Amino- and carboxyl-terminal domains of Filamin-A interact with CRMP1 to mediate Sema3A signalling Reorganization of the actin cytoskeleton is an early cellular response to various extracellular signals. Sema3A, a repulsive axon guidance molecule, induces the reorganization of actin cytoskeleton in the growth cones. Collapsin response mediator protein 1 (CRMP1) mediates the intracellular Sema3A signalling through its Ser522 phosphorylation. Here we show that UNC-33, CRMP1 C. elegans homologue, interacts with FLN-1, an actin-binding Filamin-A orthologue. In nematodes, this interaction participates in the projection of DD/VD motor neurons. CRMP1 binds both the actin-binding domain and the last immunoglobulin-like repeat of Filamin-A. The alanine mutants of Filamin-A or CRMP1 in their interacting residues suppress the Sema3A repulsion in neurons. Conversely, a phosphor-mimicking mutant CRMP1(Ser522Asp) enhances the Sema3A response. Atomic-force microscopy analysis reveals that the V-shaped Filamin-A changes to a condensed form with CRMP1(Ser522Asp). CRMP1(Ser522Asp) weakens the F-actin gelation crosslinked by Filamin-A. Thus, phosphorylated CRMP1 may remove Filamin-A from the actin cytoskeleton to facilitate its remodelling. Axon guidance is accomplished by a fine orchestrated interaction of the extracellular guidance cues and their receptors on the neural growth cones. The binding of the guidance cues to their receptors activates the intracellular signalling molecules, which regulate the actin and tubulin cytoskeleton to alter the speed and direction of the growing neurites [1] . Actin cytoskeletons, which are highly enriched in the peripheral region of growth cones, are rapidly reorganized on the environmental stimulation. Hence, the local regulation of actin filaments within the growth cones directly influences the behaviour of the neurites. Semaphorin-3A (Sema3A), one of the repulsive axon guidance cues, repels the neurites by inducing rapid rearrangement of actin cytoskeleton in the growth cones [2] . Sema3A elicits the effect through the functional receptor complex of Neuropilin-1 (NRP1) and Plexin-A (PlexA) on the growth cones [3] . Collapsin response mediator proteins (CRMPs) have been identified as the intracellular signalling molecules for Sema3A [4] . CRMPs share significant homology with UNC-33 in Caenorhabditis elegans [5] . UNC-33 is involved in the axonal outgrowth and guidance of various neurons through the regulation of tubulin dynamics and neuronal polarity in nematodes [6] , [7] , [8] . Among five members of CRMP mammalian homologues (CRMP1-5) [9] , at least CRMP1 and CRMP2 are involved in Sema3A signalling [10] . Mutant mice analysis showed that crmp1 genetically interacts with sema3a in the dendritic and synaptic development of the cortical neurons [11] . Sema3A activates cyclin-dependent kinase 5 (Cdk5), which primarily phosphorylates Ser522 in CRMP1 and CRMP2 (refs 10 , 12 ). Glycogen synthase kinase-3β (GSK3β) subsequently phosphorylates adjacent Ser/Thr residues to Ser522 in CRMP1 and CRMP2. Substitution of Ser522 with Ala in CRMP2 prevents the phosphorylation and Sema3A-induced growth cone collapse response, indicating that the Ser522 phosphorylation is an essential step for Sema3A signalling [10] . The phosphorylation of CRMP2 attenuates the tubulin polymerization and axonal elongation by interfering with the interaction of CRMP2 and tubulin heterodimers [13] . It has been shown that CRMP4 is directly associated with F-actin in vitro [14] . We have recently reported that CRMP1 is co-localized with the actin cytoskeleton in the growth cones of dorsal root ganglion (DRG) neurons [15] . Furthermore, MICAL links the signalling from Plexin to F-actin cytoskeleton through CRMPs [16] , [17] , [18] . These notions suggest that CRMPs may regulate the actin organization in Sema3A signalling. Filamin-A is a large extended actin-binding protein. Filamin-A is composed of an amino-terminal actin-binding domain (ABD) and follows tandem 24 immunoglobulin-like (Ig) repeats [19] , [20] . The Ig repeats are intervened into three domains, Ig1-15, Ig16-23 and Ig24, by two flexible hinge sequences [19] , [21] . While Ig1-15 is a linear extended chain, Ig16-23 forms a compact globular structure. The last Ig24 serves as a homophilic dimer interface. The two hinges result with Filamin-A dimer in a V-shaped flexible actin-binding protein. This makes Filamin-A crosslink with F-actin to weave three-dimensional, orthogonal networks [20] , [22] . Filamin-A interacts with numerous intracellular signalling proteins [23] . The binding of Calmodulin–Ca complex to ABD inhibits the interaction of ABD and F-actin [24] . Rho family GTPases and their regulators, such as Trio and FilGAP, bind to Ig23-24 (refs 25 , 26 , 27 ). Various transmembrane proteins including β-integrin and dopamine D2 and D3 receptors also bind to Ig16-24 of Filamin-A [28] , [29] . Filamin-A is involved in the signal transduction of several environmental cues. Mechanical stress alters the ternary structure of Filamin-A and brings the dissociation of FilGAP from the Ig23-24 repeats [30] . Filamin-A binds to a receptor tyrosine kinase Ror2 and mediates the Wnt5A-induced filopodia formation via actin reorganization [31] . Thus, Filamin-A is thought to be an important linker between extracellular signals and actin cytoskeletons. However, the mechanism of how Filamin-A connects the signalling molecules to F-actin remains elusive. In addition, functional analyses of Filamin-A in vertebrate axon guidance signalling have yet to be examined in spite of the localization of Filamin-A in the growth cones [32] . Here we show the genetic interaction between unc-33 and filamin-1 ( fln-1 ) in C. elegans . CRMP1 binds to both ABD and Ig24 of Filamin-A. Mutating the interaction residues in Filamin-A or CRMP1 reduces the interaction as well as the Sema3A-induced growth cone collapse response. In contrast, mimicking phosphorylation at Ser522 of CRMP1 with Asp augments the interaction and the Sema3A response. Furthermore, the V-shaped Filamin-A ternary structure is altered to a compact form in the presence of CRMP1(Ser522Asp). Thus, the interaction of CRMP1 and Filamin-A or of UNC-33 and FLN-1 may link the signalling from the axon guidance cues to the actin reorganization in the growing neurites. UNC-33, a C. elegans CRMP homologue, interacts with FLN-1 To identify the molecules that interact with UNC-33 and/or CRMPs, we screened 1 × 10 6 clones of a yeast two-hybrid C. elegans cDNA library with the full-length UNC-33 as the bait ( Fig. 1a ). Among the 89 positive clones obtained, 19 of them encoded a partial sequence of fln-1 (Y66H1B.2), which is orthologous to human Filamin-A [33] . The clones contained a cDNA insert encoding either amino-acid residues 1,231 to 1,522 (C) or 1,975 to 2,259 (D) of the immunoglobulin repeat (Ig) fragment of FLN-1. These FLN-1 fragments could interact with both the N-terminal region (A) and the CRMP homologous region (B) of UNC-33 in the yeast hybrid system ( Fig. 1a–c ). Alignment of FLN-1 and human Filamin-A revealed that the C-terminal 100 residues of the (C) fragment and the entire (D) fragment of FLN-1 correspond to Ig16 and Ig22-24 repeats of human Filamin-A, respectively ( Fig. 1a ). 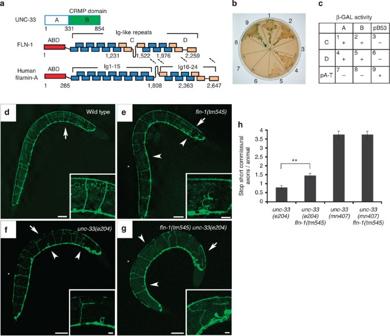Figure 1: UNC-33 interacts withC. elegansFilamin-1, FLN-1. (a) Schematic representation of UNC-33, FLN-1 and human Filamin-A. UNC-33 is composed of N-terminal region (a) and CRMP homologous region (b). Two isolated FLN-1 fragments (c,d) from yeast two-hybrid fragments are shown in orange. The C-terminal 100 residues of (c) and the entire region of (d) of FLN-1 are well conserved with Ig16 (45% identity) and Ig22-24 (40.3% identity) of human Filamin-A, respectively. ABD=actin-binding domain; Ig=immunoglobulin like repeats. (b,c) Yeast two-hybrid assay. The B and C panels represent cultured Yeast dish and a summary table, respectively. Both the N-terminal region (a, GAL4DB::UNC-33(1–331)) and the C-terminal CRMP homologous region (b, GAL4DB::UNC-33(332–854)) of UNC-33 interact with FLN-1 middle fragment (c, GAL4AD::FLN-1(1,231–1,522)) and C-terminal fragment (d, GAL4AD::FLN-1(1,975–2,259)). pGBKT7-p53 (GAL4DB::p53) and pGADT7-T (GAL4AD::T-antigen) as a positive control. (d–g) Commissural projection of DD/VD neurons in wild type,fln-1(tm545), unc-33(e204)andfln-1(tm545) unc-33(e204). DD/VD neurons were visualized byoxIs12 [unc-47::gfp]. (d) In wild type, 15–17 DD/VD axons are traversed from ventral side to dorsal side. (e) Infln-1(tm545), two DD/VD axons fail to reach the dorsal side (arrowheads). (f,g) Inunc-33(e204)andfln-1(tm545) unc-33(e204), several commissural axons fail to reach the dorsal side (arrowheads). Asterisk indicates gap of dorsal nerve cord. Inset, higher magnification of arrow indicated area. Scale bars, 50 and 10 μm (Inset). (h) The irregular commissural DD/VD neurons in one animal were scored. While a weak allele mutantunc-33(e204)showed the genetic augmentation withfln-1(tm545), a strong allele mutantunc-33(mn407)did not exhibit the augmentation withfln-1(tm545). Each bar represents average±s.e.m. (n=78,unc-33(e204); 84,unc-33(e204) fln-1(tm545); 78,unc-33(mn407); 101,unc-33(mn407) fln-1(tm545)). **P<0.01, unpairedT-test. Figure 1: UNC-33 interacts with C. elegans Filamin-1, FLN-1. ( a ) Schematic representation of UNC-33, FLN-1 and human Filamin-A. UNC-33 is composed of N-terminal region ( a ) and CRMP homologous region ( b ). Two isolated FLN-1 fragments ( c , d ) from yeast two-hybrid fragments are shown in orange. The C-terminal 100 residues of ( c ) and the entire region of ( d ) of FLN-1 are well conserved with Ig16 (45% identity) and Ig22-24 (40.3% identity) of human Filamin-A, respectively. ABD=actin-binding domain; Ig=immunoglobulin like repeats. ( b , c ) Yeast two-hybrid assay. The B and C panels represent cultured Yeast dish and a summary table, respectively. Both the N-terminal region ( a , GAL4DB::UNC-33(1–331)) and the C-terminal CRMP homologous region ( b , GAL4DB::UNC-33(332–854)) of UNC-33 interact with FLN-1 middle fragment ( c , GAL4AD::FLN-1(1,231–1,522)) and C-terminal fragment ( d , GAL4AD::FLN-1(1,975–2,259)). pGBKT7-p53 (GAL4DB::p53) and pGADT7-T (GAL4AD::T-antigen) as a positive control. ( d – g ) Commissural projection of DD/VD neurons in wild type, fln-1(tm545), unc-33(e204) and fln-1(tm545) unc-33(e204) . DD/VD neurons were visualized by oxIs12 [unc-47::gfp] . ( d ) In wild type, 15–17 DD/VD axons are traversed from ventral side to dorsal side. ( e ) In fln-1(tm545) , two DD/VD axons fail to reach the dorsal side (arrowheads). ( f , g ) In unc-33(e204) and fln-1(tm545) unc-33(e204) , several commissural axons fail to reach the dorsal side (arrowheads). Asterisk indicates gap of dorsal nerve cord. Inset, higher magnification of arrow indicated area. Scale bars, 50 and 10 μm (Inset). ( h ) The irregular commissural DD/VD neurons in one animal were scored. While a weak allele mutant unc-33(e204) showed the genetic augmentation with fln-1(tm545) , a strong allele mutant unc-33(mn407) did not exhibit the augmentation with fln-1(tm545) . Each bar represents average±s.e.m. ( n =78, unc-33(e204) ; 84, unc-33(e204) fln-1(tm545) ; 78, unc-33(mn407) ; 101, unc-33(mn407) fln-1(tm545) ). ** P <0.01, unpaired T -test. Full size image An fln-1 null mutant tm545 was generated by trimethylpsoralen treatment and UV irradiation [33] , [34] . As unc-33 mutants exhibited multiple axon guidance defects including DD/VD neurons [7] , DD/VD commissural projection in fln-1 ( tm545 ) was examined. Thirteen percent of the fln-1(tm545) animals exhibited misrouting of DD/VD neurons ( Fig. 1e , Table 1 ), while only 3% of the wild-type animals showed an abnormal projection ( Fig. 1d , Table 1 ). This irregular projection was rescued by the expression of FLN-1 with its own promoter in fln-1(tm545) ( Table 1 ). A weak allele mutant of unc-33 , unc-33(e204) , also exhibited a 43% commissural guidance defect of DD/VD neurons ( Fig. 1f , Table 1 ). Furthermore, the double mutant of fln-1(tm545) and unc-33(e204) increased the DD/VD irregular projection to 59% ( Fig. 1g , Table 1 ). In contrast, a strong allele mutant of unc-33 , unc-33(mn407) , did not exhibit the genetic augmentation with fln-1(tm545) in the double mutant ( Fig. 1h ). This confirms the genetic interaction of unc-33 and fln-1 . Thus, FLN-1 and its direct interaction with UNC-33 may participate in the axon guidance of DD/VD neurons. Table 1 Summary table for DD/VD commissural projection defects in mutants. Full size table Plx-2 genetically interacts with fln-1 in DD/VD projection As CRMPs are involved in the Semaphorin-Plexin signalling in vertebrates [10] , [11] , [35] , we asked whether FLN-1 participates in the Semaphorin signalling in nematodes. It has been shown that Sema2a, designated as mab-20, participates in the ventral fasciculation of DD/VD neurons [36] . In addition, several mutants, such as ptp-3 and unc-119 , exhibit premature termination (gap) and/or defasciculation of the DD/VD neurons in dorsal nerve cord [37] , [38] . We then examined the ventral, commissural and dorsal DD/VD projection in Sema2a null mutant, mab-20(ev574) , and in its receptor Plexin-2 mutant, plx-2(tm729) . We found that the gap or defasciculation defects of dorsal nerve cord in mab-20(ev574) and plx-2(tm729) , but not in wild-type animals ( Fig. 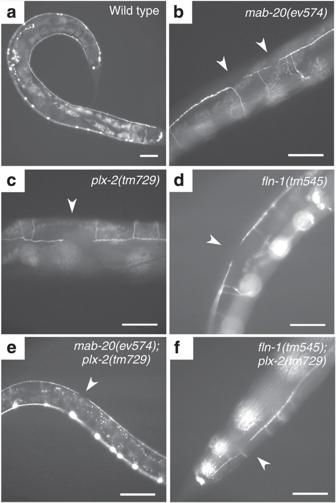Figure 2:mab-20,plx-2andfln-1mutants show premature terminations of DD/VD projection in dorsal nerve cord. (a) In wild type animals, dorsal nerve cord is single and continuous. (b–f)mab-20(ev574)(b),plx-2(tm729)(c),fln-1(tm545)(d) and their double mutant animals,mab-20(ev574); plx-2(tm729)(e) andfln-1(tm545); plx-2(tm729)(f), show gapped dorsal nerve cord. Arrowheads in the mutant panels indicate the gaps (premature terminations). Scale bar, 50 μm. 2a–c , Table 2 ). fln-1(tm545) also showed the similar phenotype (asterisk in Figs 1e and 2d , Table 2 ). plx-2(tm729) did not augment mab-20(ev574) phenotype in the double mutant ( Fig. 2e , Table 2 ), confirming the genetic interaction of these genes. Owing to the lethality of mab-20(ev574); fln-1(tm545) double mutant, we evaluated the genetic interaction of fln-1(tm545) and plx-2(tm729) . The abnormal frequency of DD/VD dorsal nerve cord in fln-1(tm545); plx-2(tm729) was the same extent as the fln-1(tm545) ( Fig. 2d,f , Table 2 ). The absence of genetic augmentation of two null mutants, fln-1(tm545) and plx-2(tm729) , suggests that FLN-1 may act as one of the downstream molecules in the Sema2a-Plexin-2 signalling in nematodes. Figure 2: mab-20 , plx-2 and fln-1 mutants show premature terminations of DD/VD projection in dorsal nerve cord. ( a ) In wild type animals, dorsal nerve cord is single and continuous. ( b – f ) mab-20(ev574) ( b ), plx-2(tm729) ( c ), fln-1(tm545) ( d ) and their double mutant animals, mab-20(ev574); plx-2(tm729) ( e ) and fln-1(tm545); plx-2(tm729) ( f ), show gapped dorsal nerve cord. Arrowheads in the mutant panels indicate the gaps (premature terminations). Scale bar, 50 μm. Full size image Table 2 Summary table for dorsal nerve cord defect of DD/VD neurons in mutants. Full size table Filamin-A is involved in Sema3A signalling Next we examined the interaction of mammalian CRMPs and Filamin-A. Human Filamin-A was co-immunoprecipitated with CRMP1, CRMP3 or CRMP4 from the transfected HEK293T cells ( Fig. 3a ). The lower expression of CRMP5 in the same condition made it impossible to confirm CRMP5–Filamin-A interaction. As CRMP1 is co-localized with actin cytoskeleton in the neurons [15] and CRMP1 is involved in Sema3A signalling [10] , [11] , we hereafter focused on clarifying the interaction between CRMP1 and Filamin-A. Co-immunoprecipitation of CRMP1 with Filamin-A from the rat E20 brain confirmed the in vivo interaction ( Fig. 3b ). Specificity of CRMP1–Filamin-A interaction was supported by the fact that GAPDH did not co-precipitate with Filamin-A ( Supplementary Fig. 1 ). During the embryonic stages, CRMP1 is predominantly expressed in both the central and peripheral nervous systems, including DRG neurons [39] . In situ hybridization revealed that Filamin-A mRNA was expressed in DRG neurons, specifically in neuronal cell bodies, sympathetic ganglia, motoneuron nuclei and the neuroepithelial layers (arrow) of the spinal cord in mouse E12 embryo ( Fig. 3c ). To assess the functional significance of the interaction between CRMP1 and Filamin-A in Sema3A signalling, the protein localization of Filamin-A, CRMP1 and F-actin in the DRG growth cones was further examined by immunostaining. Without Sema3A stimulation, confined co-localization of Filamin-A and CRMP1 was observed in the central domain of growth cones, while F-actin was localized in the peripheral region of the growth cones ( Fig. 3d , upper panels). It appears that on the addition of Sema3A, CRMP1, Filamin-A and F-actin became co-localized ( Fig. 3d , lower panels), whereas they were not in the absence of Sema3A. This suggests the functional linkage among these proteins. The co-localization of tubulin localization with the Filamin-A and CRMP1 was observed in the central domain of growth cones ( Supplementary Fig. 2a ). This co-localization increased slightly after Sema3A stimulation. 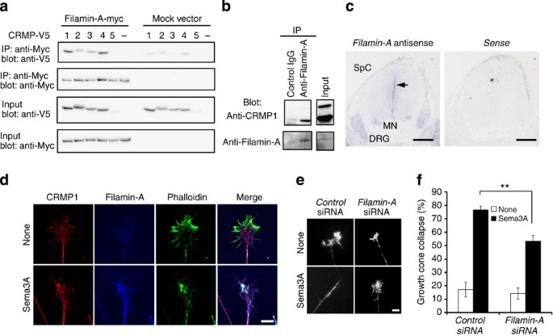Figure 3: CRMP1 interacts with Filamin-A in vertebrates. (a) Interaction of Filamin-A and CRMPs in HEK293T cells. HEK293T cells were transfected with either one of CRMP1-5-V5 expression vector together with the Filamin-A-Myc vector or a mock vector. 72 h post transfection, cells were subjected to immunoprecipitation (IP) with an anti-Myc antibody. Immunoblotting was performed as indicated. Comparing with the faint bands of CRMP1-4 in the mock vector lanes, apparent V5 blots of CRMP1, CRMP3 and CRMP4 in the Filamin-A lanes indicate the physical interaction. (b) Interaction of Filamin-A and CRMP1 in rat E20 brain. The lysates from whole-brain of E20 rats were immunoprecipitated with anti-Filamin-A mouse mAb or control mouse IgG, then probed with an anti-CRMP1 antibody. Two CRMP1 bands represent the alternate splicing isoforms. Both forms of CRMP1 are co-immunoprecipitated with Filamin-A from rat brain. (c)Filamin-AmRNA expression in mouse E12 DRG and spinal cord. Left panel, antisense probe; right panel, sense probe.Filamin-Awas expressed in DRG cell bodies (DRG) and motoneurons (MN). The neuroepithelial cell layer around the central canal in spinal cord (arrow in SpC) also expressedFilamin-A. Scale bar, 250 μm. (d) Co-localization of CRMP1, Filamin-A and F-actin in the Sema3A-stimulated DRG growth cones. Cultured mouse E12 DRG neurons were applied with or without Sema3A (0.5 U ml−1) for 5 min. The neurons were stained with anti-Filamin-A (blue) and anti-CRMP1 (red) antibodies and with Alexa488-conjugated Phalloidin (green). Without Sema3A stimulation, Filamin-A and CRMP1 were partially co-localized in the peripheral region of the growth cones. Sema3A stimulation induced the co-localization of CRMP1, Filamin-A and F-actin in the growth cones. Scale bar, 10 μm. (e,f) Suppression of Sema3A-induced collapse response ofFilamin-AsiRNA-transfected neurons. (e) The panels indicate the growth cone morphology with or without Sema3A (5 U ml−1) in mouse E12 DRG neurons transfected withFilamin-Aor control siRNA. Growth cones were stained with Alexa488-Phalloidin. Scale bar, 10 μm. (f) Scored graph. White and black bars indicate no stimulation and Sema3A (5 U ml−1) stimulation, respectively. Each bar represents average±s.e.m. (n=5 from more than three independent cultures). **P=0.003, unpairedT-test. Figure 3: CRMP1 interacts with Filamin-A in vertebrates. ( a ) Interaction of Filamin-A and CRMPs in HEK293T cells. HEK293T cells were transfected with either one of CRMP1-5-V5 expression vector together with the Filamin-A-Myc vector or a mock vector. 72 h post transfection, cells were subjected to immunoprecipitation (IP) with an anti-Myc antibody. Immunoblotting was performed as indicated. Comparing with the faint bands of CRMP1-4 in the mock vector lanes, apparent V5 blots of CRMP1, CRMP3 and CRMP4 in the Filamin-A lanes indicate the physical interaction. ( b ) Interaction of Filamin-A and CRMP1 in rat E20 brain. The lysates from whole-brain of E20 rats were immunoprecipitated with anti-Filamin-A mouse mAb or control mouse IgG, then probed with an anti-CRMP1 antibody. Two CRMP1 bands represent the alternate splicing isoforms. Both forms of CRMP1 are co-immunoprecipitated with Filamin-A from rat brain. ( c ) Filamin-A mRNA expression in mouse E12 DRG and spinal cord. Left panel, antisense probe; right panel, sense probe. Filamin-A was expressed in DRG cell bodies (DRG) and motoneurons (MN). The neuroepithelial cell layer around the central canal in spinal cord (arrow in SpC) also expressed Filamin-A . Scale bar, 250 μm. ( d ) Co-localization of CRMP1, Filamin-A and F-actin in the Sema3A-stimulated DRG growth cones. Cultured mouse E12 DRG neurons were applied with or without Sema3A (0.5 U ml −1 ) for 5 min. The neurons were stained with anti-Filamin-A (blue) and anti-CRMP1 (red) antibodies and with Alexa488-conjugated Phalloidin (green). Without Sema3A stimulation, Filamin-A and CRMP1 were partially co-localized in the peripheral region of the growth cones. Sema3A stimulation induced the co-localization of CRMP1, Filamin-A and F-actin in the growth cones. Scale bar, 10 μm. ( e , f ) Suppression of Sema3A-induced collapse response of Filamin-A siRNA-transfected neurons. ( e ) The panels indicate the growth cone morphology with or without Sema3A (5 U ml −1 ) in mouse E12 DRG neurons transfected with Filamin-A or control siRNA. Growth cones were stained with Alexa488-Phalloidin. Scale bar, 10 μm. ( f ) Scored graph. White and black bars indicate no stimulation and Sema3A (5 U ml −1 ) stimulation, respectively. Each bar represents average±s.e.m. ( n =5 from more than three independent cultures). ** P =0.003, unpaired T -test. Full size image To elucidate the functional role of Filamin-A in Sema3A signalling, the knockdown effect of Filamin-A on Sema3A-induced growth cone collapse response was examined. Transfection of three different Filamin-A siRNAs to mouse neuroblastoma Neuro2A cells or mouse DRG neurons reduced Filamin-A expression ( Supplementary Fig. 2b, c ). The neurons transfected with a mixture of the Filamin-A siRNAs were less sensitive to Sema3A stimulation ( Fig. 3e,f ). This suppression was rescued by the overexpression of human Filamin-A ( Supplementary Fig. 2d,e ). Furthermore, dual knockdown of CRMP1 and Filamin-A augmented the suppression effect of CRMP1 single knockdown on Sema3A response ( Supplementary Fig. 2g ). These results indicate that Filamin-A is involved in the intracellular signalling of Sema3A-induced growth cone collapse response. CRMP1 binds N-terminal ABD and C-terminal Ig24 of Filamin-A Filamin-A is a large protein, which consists of several different domains. Therefore, determination of the specific CRMP1 binding sites on Filamin-A would facilitate the functional analyses of the interaction. Six fragments of human Filamin-A, ABD, Ig1-5, Ig6-10, Ig11-15, Ig16-20 and Ig21-24, were bacterially expressed and purified ( Supplementary Fig. 3a ). Dot blot assay with the recombinant proteins revealed that CRMP1 bound to ABD and to a lesser extent to Ig6-10 and Ig21-24 ( Fig. 4a ). The interaction of CRMP1 and Ig21-24 correlates with the interaction of the C-terminal region of FLN-1 and UNC-33 ( Fig. 1b,c ). ABD comprises two calponin homology domains, CH1 and CH2. Within the ABD and Ig21-24, CRMP1 bound to the CH1, Ig24 and to a lesser extent to Ig23 ( Fig. 4a ). Solid-phase binding assay estimated the dissociation constant of ABD and Ig24 to CRMP1 as 1.54±0.224 μM ( n =5) and 1.47±0.499 μM ( n =5), respectively ( Supplementary Fig. 3b, c ). As ABD is the effector domain of Filamin-A, we further examined the CRMP1–ABD interaction. Deletion of the 80 to 110 residues from CH1 subdomain reduced the interaction with CRMP1 ( Supplementary Fig. 3d ). Scanning in this region with alanine mutation to attenuate side chain interactions, an ABD mutant substituted His93-Arg96 residues to alanine, ABD(H93A-R96A), and also reduced CRMP1 interaction ( Fig. 4b ). Solid-phase binding assay indicated that full-length Filamin-A wild type interacted with CRMP1 with a K d of 0.0859±0.008 μM ( n =7) while Filamin-A(H93A-R96A) mutant reduced binding to CRMP1 with a K d of 0.699±0.181 μM ( n =4) ( Fig. 4c ). According to the crystal structure of ABD (3HOP) [40] , the side chains of Gln95 and Arg96 protrude from the molecular surface ( Fig. 4d ). To verify the physical interaction in nematodes, dot blot assay with purified UNC-33 and FLN-1 fragments was performed. CRMP1 homologous region 332-854 of UNC-33 bound to both ABD and Ig19-20 of FLN-1 ( Supplementary Fig. 3e, f ). However, alanine substitution of the aligned residues (Phe75-Lys78) of FLN-1 ABD to His93-Arg96 of human Filamin-A did not attenuate to the interaction ( Supplementary Fig. 3f ). FLN-1 ABD may utilize other residues for the UNC-33 interface. 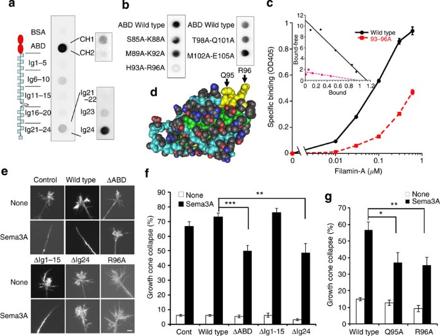Figure 4: CRMP1 interacts with both amino- and carboxyl-terminal domains of Filamin-A. (a) Dot blot assay of Filamin-A fragments. Left panel, schematic representation of Filamin-A domains. Middle panel, dot blot analysis of Filamin-A fragments. A nitrocellurose membrane blotted with 5 μg of BSA or each Filamin-A fragment was incubated with recombinant CRMP1 (1 μg ml−1). Bound CRMP1 was visualized with an anti-CRMP1 antibody. CRMP1 bound to ABD and lesser extent to Ig6-10 and Ig21-24. Right panels, dot blot analysis of ABD and Ig21-24 subdomains. CH1, subdomain of ABD, and Ig24 bound to CRMP1. (b) Determination of CRMP1-binding residues in the ABD. One microgram of wild-type ABD and various ABD alanine mutants (S85A-K88A, M89A-K92A, H93A-R96A, T98A-Q101A, M102A-E105A) were spotted onto nitrocellulose membranes. The membranes were incubated with CRMP1-V5 and bound CRMP1 was detected by an anti-V5 antibody. ABD(H93A-R96A) mutant showed weak CRMP1 interaction. (c) Specific binding of Filamin-A wild type and Filamin-A(H93A-R96A) mutant to CRMP1. Various concentrations (0–0.6 μM) of Filamin-A were incubated with solid-phased CRMP1. Filamin-A(H93A-R96A) mutant (red line) binding is reduced compared with the Filamin-A wild type (black line) binding. Dissociation constants of wild type and H93A-R96A mutants are, respectively, estimated at 0.103 and 0.626 μM from this experiment with Scatchard analysis (inset). (d) Crystal structure of CH1 subdomain of ABD (3HOP). Yellow indicates Gln95 and Arg96. The side chains of these residues protrude from the molecular surface. Space-filled view of CH1 of ABD was rendered using Cn3D (version 4.3). (e) Morphology of chick E8 DRG growth cones expressing Filamin-A mutants. Control, wildtype, ΔABD, ΔIg1-15, ΔIg24 and Filamin-A(R96A) were stimulated with 3 U ml−1Sema3A. Growth cones were stained with Alexa488-Phalloidin. (f) Quantification of Sema3A-induced collapse response. ΔABD and ΔIg24 significantly suppressed the response with Sema3A (3 U ml−1). ***P=0.0001, **P=0.003, unpairedT-test. (n=30, control; 33, wild type; 21, ΔABD; 10, ΔIg1-15; 13, ΔIg24 from more than three independent cultures). (g) Sema3A-growth cone collapse assay with Filamin-A(Q95A) and (R96A). Both single-alanine mutants significantly suppressed the growth cone collapse response with Sema3A (3 U ml−1) stimulation. *P=0.0272, unpairedT-test (n=9 from more than three independent cultures). Figure 4: CRMP1 interacts with both amino- and carboxyl-terminal domains of Filamin-A. ( a ) Dot blot assay of Filamin-A fragments. Left panel, schematic representation of Filamin-A domains. Middle panel, dot blot analysis of Filamin-A fragments. A nitrocellurose membrane blotted with 5 μg of BSA or each Filamin-A fragment was incubated with recombinant CRMP1 (1 μg ml −1 ). Bound CRMP1 was visualized with an anti-CRMP1 antibody. CRMP1 bound to ABD and lesser extent to Ig6-10 and Ig21-24. Right panels, dot blot analysis of ABD and Ig21-24 subdomains. CH1, subdomain of ABD, and Ig24 bound to CRMP1. ( b ) Determination of CRMP1-binding residues in the ABD. One microgram of wild-type ABD and various ABD alanine mutants (S85A-K88A, M89A-K92A, H93A-R96A, T98A-Q101A, M102A-E105A) were spotted onto nitrocellulose membranes. The membranes were incubated with CRMP1-V5 and bound CRMP1 was detected by an anti-V5 antibody. ABD(H93A-R96A) mutant showed weak CRMP1 interaction. ( c ) Specific binding of Filamin-A wild type and Filamin-A(H93A-R96A) mutant to CRMP1. Various concentrations (0–0.6 μM) of Filamin-A were incubated with solid-phased CRMP1. Filamin-A(H93A-R96A) mutant (red line) binding is reduced compared with the Filamin-A wild type (black line) binding. Dissociation constants of wild type and H93A-R96A mutants are, respectively, estimated at 0.103 and 0.626 μM from this experiment with Scatchard analysis (inset). ( d ) Crystal structure of CH1 subdomain of ABD (3HOP). Yellow indicates Gln95 and Arg96. The side chains of these residues protrude from the molecular surface. Space-filled view of CH1 of ABD was rendered using Cn3D (version 4.3). ( e ) Morphology of chick E8 DRG growth cones expressing Filamin-A mutants. Control, wildtype, ΔABD, ΔIg1-15, ΔIg24 and Filamin-A(R96A) were stimulated with 3 U ml −1 Sema3A. Growth cones were stained with Alexa488-Phalloidin. ( f ) Quantification of Sema3A-induced collapse response. ΔABD and ΔIg24 significantly suppressed the response with Sema3A (3 U ml −1 ). *** P =0.0001, ** P =0.003, unpaired T -test. ( n =30, control; 33, wild type; 21, ΔABD; 10, ΔIg1-15; 13, ΔIg24 from more than three independent cultures). ( g ) Sema3A-growth cone collapse assay with Filamin-A(Q95A) and (R96A). Both single-alanine mutants significantly suppressed the growth cone collapse response with Sema3A (3 U ml −1 ) stimulation. * P =0.0272, unpaired T -test ( n =9 from more than three independent cultures). Full size image Testing the dominant-negative effect of Filamin-A mutants on the Sema3A response in DRG neurons would confirm the importance of interaction domains. Compared with Filamin-A wild type, both the ABD-truncated mutant (ΔABD) and Ig24-deleted mutant (ΔIg24) suppressed the Sema3A-induced growth cone collapse response ( Fig. 4e,f ). ΔABD was localized in the central domain of the growth cone, while wild type and other mutants were co-localized with F-actin ( Supplementary Fig. 5a ). Furthermore, overexpression of Filamin-A(Q95A) or Filamin-A(R96A) also suppressed the Sema3A response ( Fig. 4e,g ). To exclude the possibility, whether the mutations in ABD reduce the ability of F-actin binding, we examined the co-sedimentation of F-actin and Filamin-A(R96A). The assay shows that the mutant retains the ability to bind F-actin as Filamin-A wild type ( Supplementary Fig. 3g, h ). Thus, the interaction of CRMP1 with both ABD and Ig24 of Filamin-A is thought to be involved in Sema3A-signalling. The middle region of CRMP1 binds to Filamin-A Dot blot assay was performed with a series of CRMP1 fragments to determine the interface region for Filamin-A ( Supplementary Fig. 4a ). A fragment from Leu225 to Met256 of CRMP1, but not any other fragments from Leu225 to Cys248 or Ala241 to Met256, bound to ABD and Ig21-24 ( Fig. 5a ). Within the 225–256 fragment, Arg245 to Asn247 are exposed to the molecular surface according to the crystal structure of mouse CRMP1 (1KCX) ( Fig. 5b ) [35] . Alanine-mutational scan of CRMP1 from Arg245 to Cys248 revealed that the single mutating Arg245, Ile246 or Asn247 reduced the binding ability to ABD ( Fig. 5c ). Solid-phase binding assay showed that Filamin-A interacted with CRMP1(N247A) with a K d of 0.178±0.020 μM ( n =4) ( Fig. 5d ), confirming the lower affinity than with CRMP1 wild type. However, alanine substitution of the aligned residues (Asn550-Ser553) of UNC-33 to Gly244-Asn247 of CRMP1 did not affect the FLN-1 binding ( Supplementary Fig. 4b ). From these results, the interface domain in UNC-33/CRMP1 may not be fully conserved among different species. The CRMP1 alanine mutants were subjected to Sema3A collapse assay in DRG neurons. Compared with the overexpression of CRMP1 wild type, CRMP1(I246A) and CRMP1(N247A) mutants significantly suppressed Sema3A response ( Fig. 5e,f ). This inhibition may not be due to the attenuation of CRMP1–Plexin-A interaction because CRMP1(N247A) retains the interaction ( Supplementary Fig. 4c ). Taken together, Ile246, Asn247 and their adjacent amino acids in CRMP1 may directly interact with Filamin-A. 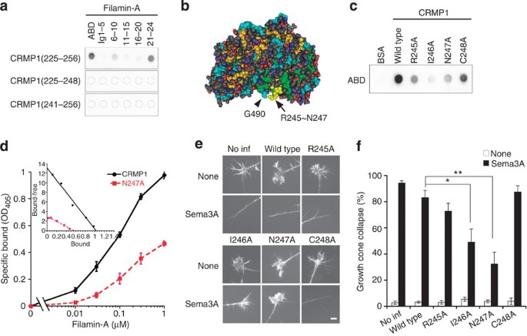Figure 5: Ile246 and Asn247 of CRMP1 are the key residues for Filamin-A interaction. (a) Binding of CRMP1 fragment 225–256 to the Filamin-A fragments. Other shorter fragments of CRMP1, 225–248 or 241–256, do not bind to the Filamin-A fragments. This indicates that the 225–256 fragment of CRMP1 comprises the minimal binding region to Filamin-A. Dashed circles indicate the spotted positions of the Filamin-A fragments. (b) Crystal structure of mouse CRMP1 (1KCX). Arrow indicates Arg245 to Asn247 residues (yellow) of CRMP1. Arrowhead indicates Gly490, a transition residue to the C-terminal region of CRMP1. Space-filled view of CRMP1 dimer was rendered using Cn3D. (c) ABD binding to CRMP1 mutants. Single-alanine mutants of CRMP1, R245A, I246A, N247A, but not C248A reduced the interaction with ABD. (d) Specific binding of Filamin-A wild type to CRMP1 or CRMP1(N247A). Various concentrations (0–1 μM) of Filamin-A were incubated with solid-phased CRMP1 wild type (black, solid line) or CRMP1(N247A) (red, dashed line). Dissociation constant of Filamin-A to CRMP1 wild type and CRMP1(N247A) were, respectively, estimated at 0.0787 and 0.191 μM from this experiment with Scatchard analysis (inset). (e) Micrograph of DRG growth cones expressing CRMP1 mutants with or without Sema3A stimulation (5 U ml−1). Growth cones were stained with Alexa488-Phalloidin. (f) Quantification of Sema3A-induced collapse response. I246A and N247A mutants suppressed Sema3A-induced growth cone collapse response. Data are mean±s.e.m. (n=10, control; 9, wildtype; 10, R245A; 10, I246A; N247A; 7, C248A from more than three independent cultures). *P=0.04, **P=0.0013, unpairedT-test. Figure 5: Ile246 and Asn247 of CRMP1 are the key residues for Filamin-A interaction. ( a ) Binding of CRMP1 fragment 225–256 to the Filamin-A fragments. Other shorter fragments of CRMP1, 225–248 or 241–256, do not bind to the Filamin-A fragments. This indicates that the 225–256 fragment of CRMP1 comprises the minimal binding region to Filamin-A. Dashed circles indicate the spotted positions of the Filamin-A fragments. ( b ) Crystal structure of mouse CRMP1 (1KCX). Arrow indicates Arg245 to Asn247 residues (yellow) of CRMP1. Arrowhead indicates Gly490, a transition residue to the C-terminal region of CRMP1. Space-filled view of CRMP1 dimer was rendered using Cn3D. ( c ) ABD binding to CRMP1 mutants. Single-alanine mutants of CRMP1, R245A, I246A, N247A, but not C248A reduced the interaction with ABD. ( d ) Specific binding of Filamin-A wild type to CRMP1 or CRMP1(N247A). Various concentrations (0–1 μM) of Filamin-A were incubated with solid-phased CRMP1 wild type (black, solid line) or CRMP1(N247A) (red, dashed line). Dissociation constant of Filamin-A to CRMP1 wild type and CRMP1(N247A) were, respectively, estimated at 0.0787 and 0.191 μM from this experiment with Scatchard analysis (inset). ( e ) Micrograph of DRG growth cones expressing CRMP1 mutants with or without Sema3A stimulation (5 U ml −1 ). Growth cones were stained with Alexa488-Phalloidin. ( f ) Quantification of Sema3A-induced collapse response. I246A and N247A mutants suppressed Sema3A-induced growth cone collapse response. Data are mean±s.e.m. ( n =10, control; 9, wildtype; 10, R245A; 10, I246A; N247A; 7, C248A from more than three independent cultures). * P =0.04, ** P =0.0013, unpaired T -test. Full size image Phosphorylation augments CRMP1-Filamin-A interaction In Sema3A signalling, Cdk5 primarily phosphorylates the Ser522 residues of CRMP1 and CRMP2 (ref. 10 ). Overexpression of a non-phosphorylated CRMP2 mutant partially blocks the Sema3A-induced growth cone collapse [10] . As the substitution of Ser/Thr with Asp/Glu tends to mimic phosphorylation, we examined whether CRMP1(S522D) mutant affects the interaction with Filamin-A. The binding assay revealed that CRMP1(S522D) bound to solid-phased Filamin-A with higher affinity (0.153±0.015 μM, n =5) than CRMP1 wild type (0.340±0.054 μM, n =6) ( Fig. 6a,b ). In contrast, the binding curve of unphosphorylated mimicking form CRMP1(S522A) was comparable to that of its wild type ( Supplementary Fig. 4d ). These findings indicate that the phosphorylation of Ser522 augments the CRMP1–Filamin-A interaction. We next examined the effect of CRMP1(S522D) on Sema3A signalling. The ectopic expression of CRMP1(S522D) in chick DRG neurons increased collapsed growth cones without Sema3A stimulation ( Fig. 6d ). This mutant also augmented the Sema3A-induced growth cone collapse response ( Fig. 6c,d ). In addition, CRMP1(S522D) formed complexes with F-actin in the central domain of the growth cones ( Supplementary Fig. 5b ). Using this CRMP1(S522D)-induced spontaneous collapse response, we asked whether Filamin-A functions as a direct downstream molecule of CRMP1 or whether Filamin-A independently mediates the collapsing signal to CRMP1. Mouse embryonic DRG neurons were primarily transfected with the Filamin-A siRNA and subsequently infected with the recombinant HSV harbouring CRMP1 wild type or CRMP1(S522D). The knockdown of Filamin-A significantly inhibited CRMP1(S522D)-induced growth cone collapse ( Fig. 6e,f ), suggesting that the interaction of phosphorylated CRMP1 and Filamin-A may regulate the growth cone morphology. 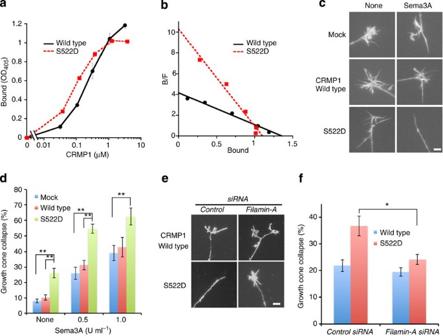Figure 6: Ser522 phosphorylation regulates CRMP1–Fimain-A interaction. (a,b) Specific binding of CRMP1 wild type and CRMP1(S522D) to Filamin-A. (a) Binding curve. (b) Scatchard analysis. Various concentrations (0–3 μM) of CRMP1 were incubated with solid-phased Filamin-A. CRMP1(S522D) mutant (red line) binding is increased compared with CRMP1 wild type (black line) binding. Dissociation constants of wild type and S522D mutants were, respectively, estimated at 0.325 and 0.107 μM from this experiment. (c) Micrograph of chick E8 DRG growth cones expressing mock vector, CRMP1 wild type or CRMP1(S522D) with or without Sema3A stimulation (0.5 U ml−1). CRMP1(S522D) overexpression induced partially collapsed growth cone without Sema3A stimulation (left bottom). Growth cones were stained with Alexa488-Phalloidin. Scale bar, 10 μm. (d) Quantification of Sema3A-induced collapse response. CRMP1(S522D) significantly augmented Sema3A response. Data are mean±s.e.m. (none,n=10, control; 11, wild type; 6, S522D; Sema3A 0.5U,n=10, control; 10, wild type; 8, S522D; Sema3A 1U,n=8, control; 10, wild type; 6, S522D from more than three independent cultures). **P<0.01, unpairedT-test. (e,f) Suppression of CRMP1(S522D)-induced morphological alteration by Filamin-A knockdown. (e) Micrograph.Filamin-ARNAi prevented the mouse E13 DRG growth cones from the CRMP1(S522D)-induced morphological alteration. Growth cones were stained with Alexa488-Phalloidin. Scale bar, 10 μm. (f) Scored graph. Data are mean±s.e.m. (n=5 from more than three independent cultures). *P<0.05, unpairedT-test. Figure 6: Ser522 phosphorylation regulates CRMP1–Fimain-A interaction. ( a , b ) Specific binding of CRMP1 wild type and CRMP1(S522D) to Filamin-A. ( a ) Binding curve. ( b ) Scatchard analysis. Various concentrations (0–3 μM) of CRMP1 were incubated with solid-phased Filamin-A. CRMP1(S522D) mutant (red line) binding is increased compared with CRMP1 wild type (black line) binding. Dissociation constants of wild type and S522D mutants were, respectively, estimated at 0.325 and 0.107 μM from this experiment. ( c ) Micrograph of chick E8 DRG growth cones expressing mock vector, CRMP1 wild type or CRMP1(S522D) with or without Sema3A stimulation (0.5 U ml −1 ). CRMP1(S522D) overexpression induced partially collapsed growth cone without Sema3A stimulation (left bottom). Growth cones were stained with Alexa488-Phalloidin. Scale bar, 10 μm. ( d ) Quantification of Sema3A-induced collapse response. CRMP1(S522D) significantly augmented Sema3A response. Data are mean±s.e.m. (none, n =10, control; 11, wild type; 6, S522D; Sema3A 0.5U, n =10, control; 10, wild type; 8, S522D; Sema3A 1U, n =8, control; 10, wild type; 6, S522D from more than three independent cultures). ** P <0.01, unpaired T -test. ( e , f ) Suppression of CRMP1(S522D)-induced morphological alteration by Filamin-A knockdown. ( e ) Micrograph. Filamin-A RNAi prevented the mouse E13 DRG growth cones from the CRMP1(S522D)-induced morphological alteration. Growth cones were stained with Alexa488-Phalloidin. Scale bar, 10 μm. ( f ) Scored graph. Data are mean±s.e.m. ( n =5 from more than three independent cultures). * P <0.05, unpaired T -test. Full size image CRMP1 alters V-shaped Filamin-A structure As CRMP1 forms homotetramer [35] and CRMP1 binds to both N- and C termini of Filamin-A ( Fig. 4a ), CRMP1 may alter the Filamin-A ternary structure by the binding. We found that CRMP1(S522D) tetramer spontaneously oligomerized and was precipitated by ultracentrifugation (arrowheads in P lanes, Fig. 7a ). Precipitated Filamin-A was increased in the presence of CRMP1(S522D) (arrow). This fact enabled us to estimate the stoichiometry of Filamin-A and CRMP1(S522D) ( Fig. 7a,b ). The Filamin-A binding curve and Scatchard plot from the co-sedimentation assay suggest that Filamin-A has both high- and low-affinity CRMP1-binding sites. The dissociation constants of these high- and low-affinity sites were estimated as 0.131 and 0.78 μM, respectively ( Fig. 7b ). Stoichiometry of the high- and low-affinity binding sites was estimated as 0.065 and 0.227 (Filamin-A/CRMP1(S522D) molar ratio), respectively ( Fig. 7b , inset). The K d for high-affinity binding sites correlated well with the K d from the solid-phase binding assay ( Figs 4c and 5d ). However, the existence of low-affinity binding characteristics from this assay may reflect flexible movement of Filamin-A and/or CRMP1 in a liquid phase. 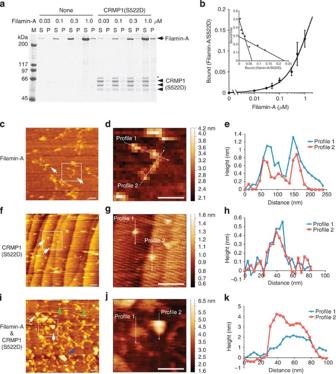Figure 7: CRMP1(S522D) induces morphological alternation of Filamin-A. (a) Co-sedimentation assay of CRMP1(S522D) and Filamin-A. Filamin-A (0.03–1 μM) was reconstituted with or without 1 μM CRMP1(S522D) and incubated at 25 °C for 1 h then ultracentrifuged. Separated specimens were subjected to 7.5% polyacrylamide gel electrophoresis and stained with Coomassie Brilliant Blue. An arrow (280 kDa) and three arrowheads (64, 60, 55 kDa) indicate Filamin-A and CRMP1(S522D), respectively. The highest CRMP1 band (64 kDa) and two lower fragments (60 and 55 kDa) represent full-length and partially cleaved products, respectively. The 66-kDa band (*) is contaminant fromE. coli. S=supernatant, P=precipitate, M=protein size marker. (b) Filamin-A binding curve and Scatchard plot. The specific binding is represented as the molar ratio of Filamin-A/CRMP1(S522D). Each point represents the average±s.e.m. of three to four independent values. Scatchard plot (inset) indicates that Filamin-A possesses high- and low-affinity binding sites of which dissociation constants are 0.131 and 0.78 μM, respectively. Stoichiometry of the high- and low-affinity binding sites is estimated as 0.065 and 0.227 (Filamin-A/CRMP1(S522D) molar ratio), respectively. (c–k) Atomic morphology and height profile of purified proteins on the sapphire (0001) surface. (c–e) Filamin-A (10 nM); (f–h) CRMP1(S522D) (40 nM); (i–k) Filamin-A (10 nM) and CRMP1(S522D) (20 nM) mixture. The specimens were scanned with Seiko Instruments Atomic force microscopy equipped with a cantilever (SI-DF3, radius 10 nm, spring constant 1.6 N ml−1) in tapping mode. (c) The Filamin-A specimen was scanned 3 × 3 μm2area and its partial view is shown. The ladders on the sapphire surfaces are atomic steps. White arrows indicate the typical molecular shape of Filamin-A. (f,i) CRMP1(S522D) and Filamin-A-CRMP1(S522D) mixture were scanned 1 × 1 μm2area. (f) CRMP1(S522D) shows small round particles. (i) The mixture image represents Filamin-A-like string (green *), small round particles (green arrows), round to oval particles (white arrows) and a large aggregation (blue arrowhead). (d,g,j) Enlarged images of boxed areas. Long arrows indicate the direction of height profiling. (d) Filamin-A branches were scanned from N-terminal to C-terminal direction. (c–j) Bar, 100 nm. (e,h,k) Height profiles. (e) One branch of Filamin-A exhibits two peaks. (h) CRMP1(S522D) particles indicate similar height and diameter. (k) Two particles in the mixture show similar diameter yet different heights. Figure 7: CRMP1(S522D) induces morphological alternation of Filamin-A. ( a ) Co-sedimentation assay of CRMP1(S522D) and Filamin-A. Filamin-A (0.03–1 μM) was reconstituted with or without 1 μM CRMP1(S522D) and incubated at 25 °C for 1 h then ultracentrifuged. Separated specimens were subjected to 7.5% polyacrylamide gel electrophoresis and stained with Coomassie Brilliant Blue. An arrow (280 kDa) and three arrowheads (64, 60, 55 kDa) indicate Filamin-A and CRMP1(S522D), respectively. The highest CRMP1 band (64 kDa) and two lower fragments (60 and 55 kDa) represent full-length and partially cleaved products, respectively. The 66-kDa band (*) is contaminant from E. coli . S=supernatant, P=precipitate, M=protein size marker. ( b ) Filamin-A binding curve and Scatchard plot. The specific binding is represented as the molar ratio of Filamin-A/CRMP1(S522D). Each point represents the average±s.e.m. of three to four independent values. Scatchard plot (inset) indicates that Filamin-A possesses high- and low-affinity binding sites of which dissociation constants are 0.131 and 0.78 μM, respectively. Stoichiometry of the high- and low-affinity binding sites is estimated as 0.065 and 0.227 (Filamin-A/CRMP1(S522D) molar ratio), respectively. ( c – k ) Atomic morphology and height profile of purified proteins on the sapphire (0001) surface. ( c – e ) Filamin-A (10 nM); ( f – h ) CRMP1(S522D) (40 nM); ( i – k ) Filamin-A (10 nM) and CRMP1(S522D) (20 nM) mixture. The specimens were scanned with Seiko Instruments Atomic force microscopy equipped with a cantilever (SI-DF3, radius 10 nm, spring constant 1.6 N ml −1 ) in tapping mode. ( c ) The Filamin-A specimen was scanned 3 × 3 μm 2 area and its partial view is shown. The ladders on the sapphire surfaces are atomic steps. White arrows indicate the typical molecular shape of Filamin-A. ( f , i ) CRMP1(S522D) and Filamin-A-CRMP1(S522D) mixture were scanned 1 × 1 μm 2 area. ( f ) CRMP1(S522D) shows small round particles. ( i ) The mixture image represents Filamin-A-like string (green *), small round particles (green arrows), round to oval particles (white arrows) and a large aggregation (blue arrowhead). ( d , g , j ) Enlarged images of boxed areas. Long arrows indicate the direction of height profiling. ( d ) Filamin-A branches were scanned from N-terminal to C-terminal direction. ( c – j ) Bar, 100 nm. ( e , h , k ) Height profiles. ( e ) One branch of Filamin-A exhibits two peaks. ( h ) CRMP1(S522D) particles indicate similar height and diameter. ( k ) Two particles in the mixture show similar diameter yet different heights. Full size image We then examined the native molecular structure of Filamin-A and the complex of Filamin-A and CRMP1(S522D) with atomic force microscopy. Filamin-A exhibits a relaxed and V-shaped structure (arrow in Fig. 7c,d ). The profile of the long axis from N-terminal to C-terminal direction indicated two peaks in one branch ( Fig. 7e ). Approximate length of one Filamin-A branch was estimated to be 148±4.0 nm ( n =24). The higher peak (1.2 nm) close to the C terminus may reflect to the compact globular structure of Ig16-23 (ref. 21 ). This length is longer than the previously reported length (80 nm) from electron micrographs [21] . The heights are also lower than the deduced dimensions from the crystal structure of ABD (3HOP, 2.6 × 3.2 × 6.3 nm) and Ig repeats (Ig10, 3RGH, 1.5 × 1.5 × 3.4 nm). These differences could be explained by different imaging methods and/or preparation of recombinant proteins. The apparent lower heights may reflect the distortion of the protein on the substrate and/or the excess force of the scanning probe. Because of the low resolution, we could not estimate the volume of Filamin-A from this analysis. CRMP1(S522D) shows a compact and round shape (arrow in Fig. 7f,g ). Two particles represented similar height profiles ( Fig. 7h ). The average of diameter and height of CRMP1(S522D) particles was 40.0±1.2 nm and 0.64±0.05 nm, respectively ( n =20). The ellipsoidal volume of CRMP1(S522D) full-length (1–572) tetramer was estimated to be ~362 nm 3 . This volume is correlating well with the estimated volume (264 nm 3 ) of truncated CRMP1 (8–490) tetramer in the crystal structure (1KCX). In contrast, small particles, string-like structures, and larger round to oval shape particles were present in the mixture of Filamin-A and CRMP1(S522D) ( Fig. 7i ). The particles (white arrows, Fig. 7i ) exhibited similar diameters (~60 nm) but different heights ( Fig. 7i–k ). Various configurations of Filamin-A and CRMP1(S522D) in the particles may bring the different heights. We measured and classified 22 particles into three height groups, 1.62, 2.43 and 3.32 nm. ( Supplementary Fig. 6a–c ). The 1.62-nm height particles showed relatively homogenous dimensions ( Supplementary Fig. 6a ), suggesting the configuration of this group might be constant. The small particles (green arrows, Fig. 7i ), of which dimensions were different from CRMP1(S522D) ( Supplementary Fig. 6d,e ), may represent the partial complex of CRMP1(S522D) and subdomains of Filamin-A. The string-like structures (green asterisk, Fig. 7i ) had similar heights to Filamin-A branches ( Supplementary Fig. 6f,g ). The presence of large aggregates (blue arrowhead in Fig. 7i , Supplementary Fig 6h,i ), which are probably the multiple complex of CRMP1(S522D) and Filamin-A, may explain the sedimentation of the complex by the ultracentrifugation ( Fig. 7a,b ). Taken together, the binding of CRMP1 alters the ternary structure of Filamin-A. CRMP1 regulates the interaction of Filamin-A and F-actin Filamin-A is an actin-crosslinking protein and form gelation with F-actin in vitro . We examined the effect of CRMP1 on this interaction by falling ball viscometry [22] , [41] . The gel formed with F-actin and Filamin-A had enough strength to support a small stainless bead on the surface ( Fig. 8a ). While the addition of CRMP1-wildtype did not affect the strength (solid line), CRMP1(S522D) reduced the viscosity and the bead fell by gravity (dashed line), suggesting that CRMP1(S522D) may interfere with the interaction of Filamin-A and F-actin. 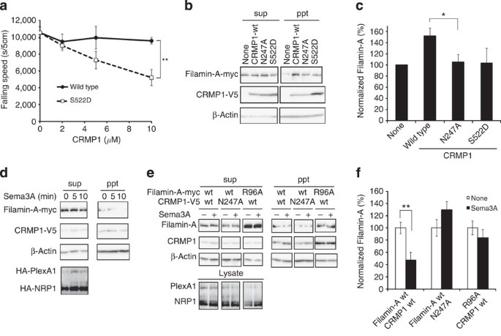Figure 8: Sema3A stimulation reduces the co-sedimentation of Filamin-A with F-actin from HEK293 cells. (a) Falling ball viscometry. The gelation of F-actin and Filamin-A with CRMP1 was examined. While addition of CRMP1 wild type did not affect the strength of Filamin-F-actin gel (solid line), CRMP1(S522D) reduced the gel viscosity and the beads placed on the gel fell by gravity (dashed line). Data are mean±s.e.m. (n=6). **P=0.0044, unpairedT-test. (b,c) Co-sedimentation of Filamin-A and F-actin from HEK293 cells expressing Filamin-A and CRMP1 mutants. Cell lysates were ultracentrifuged to precipitate F-actin and its associated proteins. Expression of CRMP1 wild type (wt) but not CRMP1(N247A) enhanced the co-precipitation of Filamin-A. (c) Scored graph. Data are mean±s.e.m. (n=6 from more than five independent experiments). *P=0.036, unpairedT-test. (d) Time course of Filamin-A co-sedimentation after Sema3A stimulation. HEK293 cells expressing Filamin-A-myc, CRMP1 wild type, HA-NRP1 and HA-PlexA1 were stimulated with Sema3A for (8 U ml−1) 0 to 10 min. Co-sedimentation of Filamin-A was decreased after 10 min Sema3A stimulation. (e,f) Attenuation by mutant proteins. HEK293 cells expressing Filamin-A, CRMP1, NRP1 and PlexA1 were stimulated with Sema3A (8 U ml−1) for 10 min. In the CRMP1 wild type (wt)-transfected cells, Sema3A stimulation reduced co-sedimentation of Filamin-A ~50% compared with the un-stimulated cells. In contrast, the cells expressing CRMP1(N247A) or Filamin-A(R96A) did not alter the Filamin-A precipitation on Sema3A stimulation. (f) Scored graph. Data are mean±s.e.m. (n=14, wild type; 10, CRMP1(N247A); 9, Filamin-A(R96A) from more than five independent experiments). **P=0.0025, unpairedT-test. Figure 8: Sema3A stimulation reduces the co-sedimentation of Filamin-A with F-actin from HEK293 cells. ( a ) Falling ball viscometry. The gelation of F-actin and Filamin-A with CRMP1 was examined. While addition of CRMP1 wild type did not affect the strength of Filamin-F-actin gel (solid line), CRMP1(S522D) reduced the gel viscosity and the beads placed on the gel fell by gravity (dashed line). Data are mean±s.e.m. ( n =6). ** P =0.0044, unpaired T -test. ( b , c ) Co-sedimentation of Filamin-A and F-actin from HEK293 cells expressing Filamin-A and CRMP1 mutants. Cell lysates were ultracentrifuged to precipitate F-actin and its associated proteins. Expression of CRMP1 wild type (wt) but not CRMP1(N247A) enhanced the co-precipitation of Filamin-A. ( c ) Scored graph. Data are mean±s.e.m. ( n =6 from more than five independent experiments). * P =0.036, unpaired T -test. ( d ) Time course of Filamin-A co-sedimentation after Sema3A stimulation. HEK293 cells expressing Filamin-A-myc, CRMP1 wild type, HA-NRP1 and HA-PlexA1 were stimulated with Sema3A for (8 U ml −1 ) 0 to 10 min. Co-sedimentation of Filamin-A was decreased after 10 min Sema3A stimulation. ( e , f ) Attenuation by mutant proteins. HEK293 cells expressing Filamin-A, CRMP1, NRP1 and PlexA1 were stimulated with Sema3A (8 U ml −1 ) for 10 min. In the CRMP1 wild type (wt)-transfected cells, Sema3A stimulation reduced co-sedimentation of Filamin-A ~50% compared with the un-stimulated cells. In contrast, the cells expressing CRMP1(N247A) or Filamin-A(R96A) did not alter the Filamin-A precipitation on Sema3A stimulation. ( f ) Scored graph. Data are mean±s.e.m. ( n =14, wild type; 10, CRMP1(N247A); 9, Filamin-A(R96A) from more than five independent experiments). ** P =0.0025, unpaired T -test. Full size image We next asked whether CRMP1 modulates the interaction of Filamin-A and F-actin in cultured cells. Filamin-A was co-sedimented with F-actin from the solubilized fractions of HEK293 cells expressing Filamin-A. Co-expression of CRMP1 wild type enhanced the Filamin-A precipitation ( Fig. 8b,c ), while CRMP1(N247A) and CRMP1(S522D), the phosphomimetic mutant of CRMP1, cancelled this augmentation. Co-sedimentation of CRMP1(S522D) with F-actin was increased compared with that of CRMP1 wild type or CRMP1(N247A). This suggests that the phosphorylation of CRMP1 may also facilitate the interaction of CRMP1 and F-actin. We then combined this co-sedimentation assay and Sema3A signalling. When the HEK293 cells expressing Filamin-A, CRMP1, NRP1 and PlexA1 were treated with Sema3A, Filamin-A co-sedimentation was decreased after 10-min stimulation ( Fig. 8d ). Filamin-A co-precipitation was reduced ~50% after Sema3A stimulation compared with the unstimulated cells ( Fig. 8e,f ). Such Sema3A-induced alteration was not observed with the cells expressing either CRMP1(N247A) or Filamin-A(R96A) mutants ( Fig. 8e,f ). These results suggest that Sema3A signalling may attenuate crosslinked F-actin cytoskeleton by enhancing CRMP1–Filamin-A interaction. FLN-1 was identified as an interactor of UNC-33. As the C-terminal region of FLN-1 bound to UNC-33 ( Fig. 1b,c ) and Ig24 of human Filamin-A bound to CRMP1 ( Fig. 3a ), the domain–domain interaction is preserved beyond species. fln-1(tm545) and unc-33(e204) mutants exhibit an irregular projection of DD/VD commissural axons. Comparing the phenotype, fln-1(tm545) exhibits a much milder defect ( Fig. 1e ) than unc-33(e204) mutant ( Fig. 1f , Table 1 ). The mild phenotype in fln-1(tm545) mutant may be due to the limited contribution of FLN-1 in DD/VD projection and/or the compensation by the other filamin isoform in C. elegans , FLN-2. The severe abnormal phenotype in unc-33 mutants may reflect the insufficient regulation of tubulin assembly [6] and/or the polarized defect [8] . fln-1(tm545) enhanced the phenotype of weak allele mutant unc-33(e204) ( Fig. 1g , Table 1 ). In contrast, fln-1(tm545) did not augment the strong allele phenotype of unc-33(mn407) ( Fig. 1h ). These results suggest that in vivo interaction of fln-1 and unc-33 participates in DD/VD commissural axon guidance. Interestingly, the mutants of Sema2a and its receptor Plexin-2, mab-20(ev574) and plx-2(tm729), are also involved in the DD/VD projection ( Fig. 2 , Table 2 ). The irregular frequency of plx-2(tm729) was milder than that of mab-20(ev574) , suggesting the participation of another receptor component in Sema2a signalling, such as LAD-2 (ref. 42 ). As plx-2(tm729) -null mutant did not augment the DD/VD phenotype of fln-1(tm545) -null mutant ( Fig. 2f , Table 2 ), these two genes are genetically interacting in DD/VD axon guidance. CRMP1 binds to ABD and Ig24 of Filamin-A. Deletion analysis of CRMP1 revealed that the middle portion (225–256) of CRMP1 is the minimal binding fragment to ABD and Ig21–24 ( Fig. 5a ). According to the CRMP1 crystal structure [35] , this fragment contains a β-sheet S15 (251–255) and an α-helix H7 (230–246), which serves as a tetramer interface by anti-parallel and homophilic interaction. As neither 241–256 nor 225–248 CRMP1 fragments interacted with ABD or Ig21-24 ( Fig. 5a ), the minimal binding fragment may dimerize to form Filamin-A interface with Asn247 and its surrounding residues. Because CRMP1 or its minimal binding fragment could bind to both ABD and Ig21-24, which are structurally unrelated, CRMP1 may recognize the limited ternary structure of these domains. Indeed, CRMP1 bound to His93-Arg96 residues in the CH1 subdomain of ABD ( Fig. 4a,c ). These residues are located in the middle of the linker between helix C and E of CH1 and are close to the actin-binding segment 2 (ref. 40 ). Interestingly, these residues are overlapped with the Calmodulin–Ca binding residues, Thr50-Arg96, in ABD [24] . Thus, as the Calmodulin–Ca complex binding to ABD reduces the interaction of Filamin-A and F-actin, CRMP1 binding to ABD may also inhibit the interaction. Filamin-A and CRMP1 forms homo-dimer and homo-tetramer in their native condition, respectively [21] , [35] . As both ABD and Ig24 of Filamin-A are capable of interacting with CRMP1, Filamin-A dimer may possess at least four binding sites. CRMP1 tetramer is also thought to possess four binding sites. Then, if the four binding sites in one Filamin-A dimer were occupied by one CRMP1 tetramer, the stoichiometry of Filamin-A/CRMP1 would become 0.5. However, the co-sedimentation assay showed that the estimated stoichiometry of Filamin-A/CRMP1(S522D) at the lower affinity was 0.227 ( Fig. 7b ). This suggests that one Filamin-A dimer may bind approximately two CRMP1(S522D) tetramers. In such a complex, at least two different binding patterns of one Filamin-A dimer and two CRMP1 tetramers may be present. 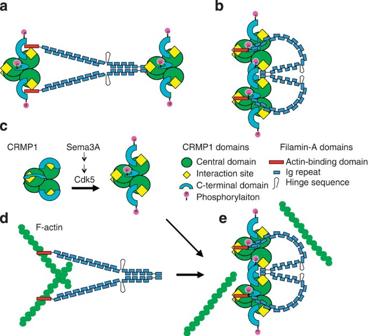Figure 9: Schematic representation of CRMP1–Filamin-A interaction in Sema3A signalling. (a,b) Two possible configurations of CRMP1 and Filamin-A complex. (a) One CRMP1 tetramer binds to either the pair of N-terminal actin-binding domain (ABD) or the pair of the C-terminal Ig24. (b) One CRMP1 tetramer simultaneously binds to ABD and Ig24. (c) Sema3A–CRMP1 signalling. Sema3A stimulation activates Cdk5, which subsequently phosphorylates the Ser522 of CRMP1. This phosphorylation facilitates the interaction of CRMP1 and Filamin-A. (d) Crosslinking F-actin by Filamin-A. Filamin-A dimer binds to F-actin through the actin-binding domain (ABD) of each branch. This brings F-actin crosslinking. (e) Removal of Filamin-A from F-actin. Formation of Filamin-A and CRMP1 complex would remove Filamin-A from F-actin in turn to weaken the cytoskeleton. Figure 9 shows the two possible configurations: (a) one CRMP1 tetramer binds to either the pair of ABD or the pair of Ig24; (b) one CRMP1 tetramer binds to ABD and Ig24. The latter (b) form may represent the oval shape particles in Filamin-A and CRMP1(S522D) mixture ( Fig. 7i ). However, CRMP family forms heterotetramers in vivo [43] . Co-immunoprecipitation assay indicates that each CRMP member has a different affinity for Filamin-A ( Fig. 3a ). Therefore, the combination of CRMP1 with other CRMP family members may attribute to the binding stoichiometry of Filamin-A. Figure 9: Schematic representation of CRMP1–Filamin-A interaction in Sema3A signalling. ( a , b ) Two possible configurations of CRMP1 and Filamin-A complex. ( a ) One CRMP1 tetramer binds to either the pair of N-terminal actin-binding domain (ABD) or the pair of the C-terminal Ig24. ( b ) One CRMP1 tetramer simultaneously binds to ABD and Ig24. ( c ) Sema3A–CRMP1 signalling. Sema3A stimulation activates Cdk5, which subsequently phosphorylates the Ser522 of CRMP1. This phosphorylation facilitates the interaction of CRMP1 and Filamin-A. ( d ) Crosslinking F-actin by Filamin-A. Filamin-A dimer binds to F-actin through the actin-binding domain (ABD) of each branch. This brings F-actin crosslinking. ( e ) Removal of Filamin-A from F-actin. Formation of Filamin-A and CRMP1 complex would remove Filamin-A from F-actin in turn to weaken the cytoskeleton. Full size image Imaging with atomic force microscopy also supports the complex formation. The larger particles appeared in the Filamin-A-CRMP1(S522D) mixture have distinct dimensions from Filamin-A or CRMP1(S522D) ( Fig. 7e,h,k ). The low height (1.62 nm) group exhibited similar dimensions ( Supplementary Fig. 6a ) and its ellipsoidal volume is calculated as 1,680 nm 3 . The volume of CRMP1(S522D) tetramer is 362 nm 3 from the averaged dimensions. Filamin-A dimer volume is estimated to be 650 nm 3 using the structural information of ABD (3HOP) and Ig10 (3RGH). Then the approximate volume of the complex, one Filamin-A dimer and two CRMP1(S522D) tetramers, would become 1,400 nm 3 , which might be close to the ellipsoidal volume of the low-height group. This may also support the stoichiometry of Filamin-A and CRMP1(S522D) in the complex obtained from the co-sedimentation assay ( Fig. 7b ). Filamin-A is an actin-crosslinking protein and forms gelation with F-actin in vitro . The gel strength was reduced in the presence of CRMP1(S522D), the phosphomimetic mutant of CRMP1 ( Fig. 8a ). In the cell culture system, overexpression of CRMP1 wild type enhanced the interaction of Filamin-A and F-actin, while CRMP1(N247A) or CRMP1(S522D) cancelled this augmentation ( Fig. 8b,c ). Activation of Sema3A-Plexin-A signalling also reduced the interaction ( Fig. 8d–f ). Taken together, Sema3A signalling induces phosphorylated CRMP1 ( Fig. 9c ), which may remove Filamin-A from the F-actin cytoskeleton crosslinked with Filamin-A ( Fig. 9d,e ). The F-actin may be further depolymerized with MICAL [16] , [17] . However, this model may not fully explain the localization of CRMP1, Filamin-A and F-actin in the growth cones. In the un-stimulated growth cones, limited co-localization of Filamin-A and F-actin was observed ( Fig. 3d upper lanes). Sema3A stimulation induced the co-localization of CRMP1, Filamin-A and F-actin in the central domain of growth cones ( Fig. 3d lower lanes). As these confocal images are the acute phase (5 min) of Sema3A stimulation, Filamin-A and F-actin may be transiently co-localized before their dissociation. Precise behaviour of these molecules in the Sema3A-treated growth cones would be investigated by live-imaging with the fluorescent-fusion proteins in the future. Our study revealed that Filamin-A RNAi-knockdown suppressed the Sema3A-induced growth cone collapse response in DRG neurons ( Fig. 3e,f ). The overexpression of Filamin-A(Q95A), Filamin-A(R96A) or CRMP1(N247A) mutants, of which the interaction residues are mutated with alanines, inhibited the Sema3A-collapse response in DRG neurons ( Figs 4e,g and 5e,f ). In addition, Filamin-A co-sedimentation with F-actin was reduced after Sema3A stimulation with the HEK293 cells expressing Sema3A receptors and CRMP1 wild type, but not with the cells expressing CRMP1(N247A) or Filamin-A(R96A) ( Fig. 8d–f ). Thus, Sema3A signalling may utilize these residues for the interface of CRMP1–Filamin-A interaction. The C-terminal Ig24 of Filamin-A also interacts with CRMP1 ( Fig. 4a , Supplementary Fig. 3c ). Overexpression of Ig24-deleted Filamin-A mutant suppressed Sema3A-induced collapse response ( Fig. 4e,f ). However, this dominant-negative effect could be attributed either by insufficient CRMP1 binding or by the incapable dimerization because Ig24 is the dimer-interface of Filamin-A. Determination and point-mutational analysis of CRMP1-binding residues in Ig24 would clarify this notion. Sema3A stimulation enhances the phosphorylation of Ser522 in C-terminal regions of CRMP1 and CRMP2 in growth cones [10] . The C-terminal phosphorylation of CRMP2 by Cdk5 and GSK3β attenuates the interaction between CRMP2 and tubulin heterodimer [10] , [13] . Lin et al. reported that the phosphorylation of CRMP1/2 C terminal by GSK3β attenuates the interaction of CRMP1/2 and microtubules [44] . We found that CRMP1(S522D), a Cdk5-phosphor mimicking mutant, bound Filamin-A with higher affinity than CRMP1 wild type ( Fig. 6a,b ). CRMP1(S522D) also potentiated Sema3A-induced growth cone collapse ( Fig. 6c,d ). At least two possible mechanisms could explain the augmentation of CRMP1(S522D) and Filamin-A interaction. Phosphorylated Ser522 would directly interact with Filamin-A. Alternatively, the C-terminal domain of CRMP1 would cover the Filamin-A-binding residues (Arg245-Asn247) that locate the adjacent C-terminal transitional residue (Gly490) ( Fig. 5b ). Then, the phosphorylation of Ser522 might alter the C-terminal ternary structure in turn to expose the Filamin-A-binding sites. These possibilities would be further studied in the structural analysis of CRMP1(S522D) complex with Filamin-A ABD or Ig24. It has been shown that Sema3A acts as an endogenous inhibitor for nerve regeneration [45] . Our data suggest that CRMP1-Filamin-A interaction mediates Sema3A signalling. We also determined the specific amino-acid residues in CRMP1, Arg245-Asn247, for Filamin-A interaction. Development of small compounds specifically bound to these residues would promise a novel approach for axonal regeneration. Animals C57B6/J mice and Wistar rats were purchased from Japan SLC (Hamamatsu, Japan). Chicken eggs were purchased from Yamagishism (Gunma, Japan) and incubated at 37 °C for 7–8 days with periodic rotation. All procedures utilizing animal specimens were performed according to the guidelines in the Institutional Animal Care and Use Committee of the Yokohama City University School of Medicine. Throughout the experimental procedures, all efforts were made to minimize the number of animals used and their suffering. Yeast two-hybrid screening Primers are listed in the Supplementary Table 1 . The C. elegans cDNA library in pACT vector (gift from R. Barstead) for two-hybrid screening was utilized. UNC-33 coding region (2.6 kbp) was amplified with UNC-33-5′ and UNC-33-3′ primers from a reverse transcribed C. elegans mRNA template. The fragment was cloned into pGBKT7 (Clontech, Mountain View, CA, US) to generate pGBKT7-UNC-33. Yeast strain AH109 was co-transfected with the pACT library and pGBKT7-UNC-33. Library screening and α-galactosidase assays were performed as described in Yeast Protocols Handbook (Clontech). C. elegans strains, cultures and phenotypic analyses Bristol strain N2 was used as the standard wild type strain. fln-1(tm545) was generated by UV and trimethylpsoralen treatment [33] , [34] . In tm545 , 263 bp in the junction of exon 3 and following intron of the fln-1 gene are deleted [33] . This brings premature 96 amino-acid protein product, which is insufficient to form a functional ABD (270 residues). Thus, tm545 thought to be a null mutant of fln-1 . unc-33(e204) and unc-33(mn407) was provided from Caenorhabditis Genetics Center. mab-20(ev574) and plx-2(tm729) were provided by JG Culotti and by S Takagi, respectively. To visualize DD/VD neurons, tm545 and other mutants were intercrossed with oxIs12[unc47::GFP] [46] . Phenotypic analysis of fln-1(tm545) , unc-33(e-204) , and the double mutants was followed. The animals in which any DD/VD neurons failed to reach dorsal side were scored as ‘irregular’. Seventy-three to 120 animals from each strain were analysed. The number of failed DD/VD commissures in one animal was also scored for the analysis of fln-1(tm545) and unc-33 interaction. The projection of DD/VD neurons in dorsal nerve cord was analysed for mab-20(ev574) , plx-2(tm729) , mab-20(ev574); plx-2(tm729) and plx-2(tem729); fln-1(tm545) mutants. Gap (premature termination) and defasciculation (including premature bifurcation) of dorsal nerve cord were scored as irregular projection. Premature termination of caudal projection of dorsal nerve cord, which does not reach above DD6 cell body, was also treated as gap phenotype. Images of DD/VD projection in these strains were captured using a laser scanning microscope (LSM510, Carl Zeiss) with an objective at × 20. Some images were taken through × 40 objective lenses equipped with an AxioPlan 2 microscope (Carl Zeiss) and a Spot-2e CCD camera (Spot, Sterling Heights, MI). C. elegans transgenics The 4.3-kbp promoter region of fln-1 gene was amplified with two primers (fln-1-Prom-5′ and fln-1-Prom-3′) from N2-genomic DNA. The Fln-1 ORF fragment (6.8 kbp) was also amplified with two primers (fln-1-ORF5′ and fln-1-ORF3′) by RT-PCR. Both fragments were cloned into pPD95.75 to generate pFln-1p::Fln-1 . Extrachromosomal arrays of ghEx36 and ghEx37 were generated by co-microinjection of the DNAs [ pFln-1p::Fln-1 (10 ng ml −1 ), pmyo-2P::mRFP (10 ng ml −1 ) and pBluescript SK+(80 ng ml −1 )] into adult N2 gonads [47] . Transformants were selected based on the mRFP expression in the pharynx. ghEx36 and ghEx37 were intercrossed with fln-1(tm545);oxIs12 . The DD/VD projection in fln-1(tm545);oxIs12;ghEx36 and fln-1(tm545);oxIs12;ghEx37 was scored. For unc-33 rescue experiments, unc-33 gene expression plasmid, pKK1510 unc-33lms , was utilized [48] . Extrachromosomal arrays of ghEx59 and ghEx60 were generated by co-microinjection of the DNAs [ pKK1510 (10 ng ml −1 ), pmyo-2P::mRFP (10 ng ml −1 ) and pBluescript SK+(80 ng ml −1 )] into adult unc-33(e204) gonads. The DD/VD commissural projection in unc-33(e204);oxIs12;ghEx59 and unc-33(e204);oxIs12;ghEx60 was scored. Plasmid construction Primers are listed in the Supplementary Table 1 . Using human Filamin-A (hFlnA) cDNA (FLJ00343) as a template, the entire coding region of hFlnA was amplified with hFlnA-f and hFlnA-r primers. Deletion mutants of ABD (ΔABD) and Ig24 (ΔIg24) were PCR-amplified with hFlnA-276f and hFlnA-r and with hFlnA-f and hFlnA-2557r, respectively. These fragments were cloned into pcDNA3.1/ myc -His A (Invitrogen). Deletion of Ig1-15 mutant (ΔIg1-15) was PCR-amplified with hFlnA-274r and hFlnA-1765f primers using pcDNA3.1-hFlnA-mycHis as a template. The coding fragment of ABD was amplified with hFlnA-2f and hFlnA-274r and cloned into pGEX6P1 (GE healthcare, US). pGEX6P vectors containing Ig1-5, Ig6-10, Ig11-15, Ig16-20, Ig21-24 and Ig24 were also constructed. The truncation and point mutations were introduced to the pGEX6P-ABD or pcDNA3.1-hFlnA-mycHis. Rat CRMP1 (rCRMP1)-coding region was amplified with rCRMP1-1f and rCRMP1-572-V5r and cloned into pGEX6P1. CRMP1-truncated fragments were PCR-amplified with the listed primers and cloned into pGEX6P-V5. Single-amino-acid mutation of rCRMP1 from Arg245 to Cys248 with alanine was introduced into pGEX6P-rCRMP1-V5 with the listed primers using QuickChange Multi Site-Directed Mutagenesis Kit (Stratagene, La Jolla, CA, US). Substitution of Ser522 to Asp (S522D) in CRMP1 was introduced with rCRMP1-521r and rCRMP1-S522Df primers by PCR. The coding fragment of mutated CRMP1 or Filamin-A was transferred to pHSV vector for the preparation of recombinant herpes simplex viruses. In brief, 2-2 cells were transfected with one of the constructed pHSV vectors and subsequently infected with IE2 defective herpes-simplex virus (5dl1.2). Mock virus was prepared with the pHSV vector without any insertion. All mutations were confirmed by DNA sequencing. Immunoprecipitation HEK293T cells (1.6 × 10 5 cells/well in a six-well dish) were transfected with the expression vectors of Filamin-A-Myc and either one of V5-tagged CRMP1, CRMP2, CRMP3, CRMP4 or CRMP5 using FuGENE 6 (Roche, Meylan, France). After 3 days incubation, the cells were rinsed once with phosphate-buffered saline (pH 7.4) (PBS) and lysed in 500 μl of lysis buffer (20 mM Tris HCl pH7.4, 150 mM NaCl, 0.5 mM Na 3 VO 4 , 1 mM NaF, 5 mM EDTA, 50 μM p-APMSF, 1% Triton X-100). The lysates were centrifuged at 20,000 × g for 15 min at 4 °C. The supernatants were incubated with an anti-Myc polyclonal antibody (1 μg) for 16 h at 4 °C, followed by further incubation with Protein G (GE, Little Chalfont, UK) for 2 h at 4 °C. After washing three times with the lysis buffer, the samples were analysed by immunoblot with anti-V5 or anti-Myc antibodies. Whole-brains from E20 rat embryos were homogenized in the lysis buffer. The lysates were centrifuged at 20,000 × g for 15 min and the supernatants were diluted to 1 mg ml −1 concentration with the buffer. The lysate (1 mg) was mixed with anti-Filamin-A mouse mAb (2 μg) for 2 h at 4 °C, followed by further incubation with Protein G for 2 h at 4 °C. Precipitated Filamin-A and CRMP1 were probed with anti-Filamin-A mouse mAb or anti-CRMP1 hamster mAb, respectively. Uncropped images are shown in Supplementary Fig. 7 . Antibodies used in this study and their dilutions are listed in Supplementary Table 2 . In situ hybridization The N-terminal region (residues 1–275) of mouse Filamin-A was PCR-amplified with mFlnA-1f and mFlnA-275r primers from reverse-transcribed mouse brain cDNA template and cloned into pBlueScriptSK+. Digoxigenin-labelled mouse Filamin-A cRNA probes were prepared from this construct using T7 or T3 RNA polymerase. Horizontal cryostat sections (16-μm thick) at cervical level from ICR mouse E12 embryos were hybridized with the probes. Bound probes were visualized with an alkaline phosphatase-conjugated anti-Digoxigenin antibody. DRG culture and growth cone collapse assay Eight-well tissue culture plates (Nunc, Rochester, NY, US) were coated with 100 μg ml −1 poly- L -lysine and 8 μg ml −1 mouse laminin. The dorsal root ganglia (DRG) were dissected from E8 chick or from E12–16 mouse (C57B6/J) embryos. Chick DRG explants were placed in a well containing 250 μl of F12 ham supplemented with 5% FBS, 16.7 ng ml −1 2.5S NGF, 50 U ml −1 Penicillin and 50 μg ml −1 Streptomycin. The dominant-negative effect was examined with the infection of the recombinant herpes-simplex viruses harbouring the CRMP1 or Filamin-A mutants to the DRG explants. Negative control was treated with the infection of the mock virus. The explants were cultured at 37 °C for 1 day unless otherwise noted. Expression of these mutants in DRG neurons was confirmed by anti-myc or anti-V5 immunocytochemistry ( Supplementary Fig. 5 ). Mouse DRG explants were placed in a well containing 250 μl of mouse DRG medium, which consists of NeuroBasal supplemented with 2% B-27 (Invitrogen), 0.5 mM L -glutamine, 16.7 ng ml −1 2.5S NGF, 50 U ml −1 Penicillin and 50 μg ml −1 Streptomycin. Growth cone collapse assays were performed with purified recombinant chick Sema3A [4] . The explants were incubated with Sema3A at 37 °C for 20 min followed by fixation. Growth cones were stained with Alexa488-phalloidin (Invitrogen). The growth cones without lamellipodia or filopodia were scored as collapsed. One Unit per ml concentration of Sema3A induced 50% collapsed growth cones of chick E7 DRG neurons. Growth cone images were captured through × 40 objective lenses equipped with an Olympus IX-70 microscope and a Spot-2e CCD camera. siRNA transfection Three different mouse Filamin-A siRNAs (sc-35375 A, B, C) were purchased from Santa Cruz Biotech. These siRNAs equally suppressed Filamin-A expression in Neuro2A cells ( Supplementary Fig. 2b ). Mouse CRMP1 siRNA mixture (sc-60446) from Santa Cruz Biotech reduced CRMP1 expression in Neuro2A cells ( Supplementary Fig. 2f ). Transfection of the siRNA mixture into mouse DRG was performed with GeneSilencer Transfection Reagent (Genlantis, San Diego, CA, US) or DharmaFECT-3 (Thermo Scientific, Waltham, MA, US). In brief, 140 pmol of siRNA was mixed with 6 μl of either one of the transfection reagents in 220 μl of Neurobasal medium. The aliquot of the mixture (25 μl) was added to one well (250 μl) containing a DRG explant. After 4 h incubation at 37 °C, the medium was replaced with the fresh mouse DRG medium. The DRG explants were further incubated for 2 to 3 days [49] . Immunocytochemistry of DRG growth cones Mouse DRG explants were exposed to Sema3A (0.5 U ml −1 ) for 5 min and were fixed by adding equal volume of 4% PFA/PBS. The explants were blocked with 5% normal goat serum and 0.1% Triton X-100 in PBS for 1 h. The explants were incubated with anti-CRMP1 hamster mAb (1:500), anti-Filamin-A rabbit mAb (1:100) and Alexa488-conjugated Phalloidin (1:500) in the blocking solution at 4 °C overnight, following by incubation with Cy3-labelled anti-hamster antibody (1:1,000) and Alexa647-labeled anti-rabbit antibody (1:1,000) at RT for 1 h. Co-immunostaining with anti-tubulin mouse mAb (1:2,000) was also examined. The growth cones were analysed using Zeiss LSM510 confocal microscopy with an objective at × 63. Purification of recombinant proteins GST-fused CRMP1 and Filamin-A fragments were expressed in BL21 E. coli strain, affinity-purified with glutathione-resin and digested with PreScission protease (GE). His-tagged human Filamin-A-myc was stably expressed in HEK293 cells and affinity purified with Co-resin (TALON, Clontech). For atomic force microscopic analysis, the proteins were further purified with Sephacryl S-300 gel chromatography. Full-length Filamin-A was purified near 90% homogeneity. Dot blot assay Dot blot assay was performed according to standard procedures [50] . In brief, purified Filamin-A fragments (0.5–5 μg) were spotted onto a nitrocellurose membrane. The membrane was incubated with CRMP1-V5 (1–5 μg ml −1 ) in the dot blot buffer containing 20 mM Hepes-NaOH pH7.4, 150 mM NaCl, 0.5% NP40 and 1 mM DTT at RT for 2 h. The membrane subsequently reacted with anti-V5 mouse mAb and HRP-conjugated anti-mouse antibodies. Bound probes were detected by chemiluminescence. Solid-phase binding assay Purified CRMP1 (0.1 mg ml −1 in PBS) was absorbed to a 96-well plate (Greiner, Frickenhausen, Germany). After blocking with PBS/5% FBS, the wells were incubated with various concentrations of purified Filamin-A (0–1 μM) in the buffer containing PBS/5% FBS at RT for 2 h. The plate was washed with PBS five times and subsequently incubated with anti-Filamin-A mouse mAb, biotinylated-anti-mouse IgG antibody and VECTASTAIN ABC-AP KIT (Vector, 3.6 μl A+3.6 μl B in 1 ml PBS/5% FBS). Bound probes were visualized with substrate p-Nitrophenyl Phosphate (Sigma) and the absorbance (405 nm) of each well was measured by a plate reader. Specific binding was estimated by subtracting the values of uncoated wells from the values of CRMP1-coated wells. Co-sedimentation assay Purified CRMP1(S522D) was ultracentrifuged at 163,000 × g at 25 °C for 30 min to separate aggregated proteins. Various concentrations of Filamin-A (0.001 to 1 μM) were reconstituted with or without 1 μM CRMP1(S522D) in the reconstitution buffer (50 μl) containing 40 mM Tris HCl pH8.0, 5 mM MgCl 2 , 125 mM NaCl and 0.2 mM DTT, then incubated at 25 °C for 1 h. Filamin-A (0.03 to 1 μM) and actin (9.6 μM) reconstitution was also performed in the same buffer supplemented with 0.5 mM ATP. The samples were ultracentrifuged at 163,000 × g for 30 min at 25 °C. Separated specimens were subjected to 7.5% polyacrylamide gel electrophoresis and stained with Coomassie Brilliant Blue. The stained gel was scanned with a film scanner (EPSON GT-X970) as 16bit white and black TIFF. The density of stained Filamin-A and CRMP1(S522D) bands was analyzed with Fiji, an Image-J derivative program [51] . Specific binding was given by the subtraction of Filamin-A density without CRMP1 from the density with CRMP1(S522D). Atomic force microscopy Purified Filamin-A (1 μM) and CRMP1-S522D (2 μM) were mixed in the PBS/Ca buffer (Phosphate buffered serine pH7.4, 0.9 mM CaCl 2 ) and incubated on ice for 3 h. The complex was 100-fold diluted with PBS/Ca and immediately adsorbed on single-crystalline sapphire (0001) surface consisted of atomic steps and atomically flat terraces at 20 °C for 15 min. Filamin-A or CRMP1(S522D) were, respectively, diluted to 10 or 40 nM with PBS/Ca and absorbed. Scanning of purified proteins was performed as described previously [52] . In brief, the specimens were soaked in PBS/Ca and were scanned in the selected area (1 × 1 μm or 3 or 3 μm) on the surface with Seiko Instruments Atomic force microscopy (E-sweep) equipped with a cantilever (SI-DF3, radius 10 nm, spring constant 1.6 N m −1 ) in a tapping mode. Obtained AFM images were analysed with Gwyddion software [53] . Diameters or lengths were corrected by the subtraction of the lateral length from the measured length. Dimensions of protein structure were calculated with MacPyMOL. Molecular volume from crystal information was estimated with VADAR web server [54] . The volume of Filamin-A dimer (650 nm 3 ) was estimated by the summation of the volumes of ABD(3HOP) and Ig10(3RGH), 33.0 and 12.1 nm 3 , respectively. Falling ball viscometry Gelation was determined using a miniature falling ball viscometer [41] . In brief, actin polymerization was initiated by the addition of 24 μM actin monomer in the presence of 0.24 μM Filamin-A and different concentrations (0 to 10 μM) of CRMP1 wild type or S522D in the buffer (20 mM Tris-HCl pH7.4, 100 mM KCl, 2 mM MgCl 2 , 0.5 mM EGTA, 0.5 mM ATP, 0.02% NP-40). The mixtures were drawn into 100-μl capillary tubes then the tubes were vertically placed. After 1 h incubation at RT, a stainless steel ball (0.7 mm diameter) was placed on the gel surface and its falling speed was monitored. Co-sedimentation of Filamin-A and F-actin from HEK293 cells HEK293 cells (2.5 × 10 5 cells) stably expressing Myc-tagged Filamin-A wild type or Filamin-A(R96A) mutant were transfected with the expression vectors HA-NRP1, HA-PlexA1 and CRMP1-V5 or CRMP1(N247A)-V5. After 2 days incubation, cells were stimulated with Sema3A (8 U ml −1 ) for 10 min. Cells were lysed with 500 μl of the lysis buffer and centrifuged 500 × g for 5 min at 4 °C to remove nuclei. Then the lysate was ultracentrifuged 163,000 × g for 30 min at 4 °C. Separated specimens were subjected to 7% polyacrylamide gel electrophoresis and immunoblotted with anti-Myc, anti-V5 and anti-β-actin mAbs. The density of Filamin-A band was analysed with ImageJ. In each experiment, the average of Filamin-A density of un-stimulated samples was normalized as 100%. Then the relative alteration of stimulated specimens was scored. Uncropped images are shown in Supplementary Fig. 7 . Statistical analysis The statistical significance was assessed by Fisher’s exact probability test, χ 2 -test or two-tailed unpaired Student’s T -test. Differences were considered to be significant at P <0.05. All data are presented as mean±s.e.m. The sample sizes were similar to those used in previous publications. How to cite this article: Nakamura, F. et al. Amino- and carboxyl-terminal domains of Filamin-A interact with CRMP1 to mediate Sema3A-signalling. Nat. Commun. 5:5325 doi: 10.1038/ncomms6325 (2014).